OXR1 maintains the retromer to delay brain aging under dietary restriction Dietary restriction (DR) delays aging, but the mechanism remains unclear. We identified polymorphisms in mtd , the fly homolog of OXR1 , which influenced lifespan and mtd expression in response to DR. Knockdown in adulthood inhibited DR-mediated lifespan extension in female flies. We found that mtd / OXR1 expression declines with age and it interacts with the retromer, which regulates trafficking of proteins and lipids. Loss of mtd / OXR1 destabilized the retromer, causing improper protein trafficking and endolysosomal defects. Overexpression of retromer genes or pharmacological restabilization with R55 rescued lifespan and neurodegeneration in mtd -deficient flies and endolysosomal defects in fibroblasts from patients with lethal loss-of-function of OXR1 variants. Multi-omic analyses in flies and humans showed that decreased Mtd/OXR1 is associated with aging and neurological diseases. mtd/OXR1 overexpression rescued age-related visual decline and tauopathy in a fly model. Hence, OXR1 plays a conserved role in preserving retromer function and is critical for neuronal health and longevity. Aging is a leading contributor to cognitive decline, but dietary restriction (DR) delays aging across species and slows the progression of neurodegenerative diseases [1] ; however, the mechanisms that mediate the protective effects of DR in the brain are not fully understood [2] . Additionally, factors such as natural genetic variation greatly influence response to DR, leading to the concept of precision nutrigeroscience to understand how differences between individuals and across tissues modulate responses to diet and influence healthspan and lifespan [2] . We previously used the Drosophila Genetic Reference Panel (DGRP) [3] to better understand the genetic effectors of DR-based lifespan response [4] , and in this current study, we focus on polymorphisms in the gene mustard ( mtd ), which associate with DR-dependent longevity. Genetic variants in the human homolog of mtd , Oxidation Resistance 1 (OXR1) , are associated with cerebellar atrophy, hypotonia, language delay, and seizures [5] , and its overexpression improves survival in a mouse model of amyotrophic lateral sclerosis (ALS) [6] . Despite the protective properties of OXR1, its biochemical mechanism remains unknown. Here, we identify the dietary and genetic factors which regulate mtd / OXR1 and demonstrate its necessity for the maintenance of the retromer complex, which is a heteropentameric complex of proteins necessary for recycling transmembrane proteins and lipids from endosomes to the trans -Golgi network or the cell membrane [7] , [8] . We further show that mtd / OXR1 regulates a network of genes that are essential for protection against brain aging and neurodegenerative diseases across flies and humans. Neuronal expression of mtd is required for lifespan extension upon DR To identify regulators of the protective effects of DR, we measured lifespan under ad libitum (AL, 5% yeast) or DR (0.5% yeast) conditions in female flies from 160 DGRP strains [4] . We identified genetic variants in five genes which significantly associated with extreme longevity upon DR (Supplementary Data 2 ). Of these genes, only Ferredoxin ( Fdxh ) and mustard ( mtd ) have human orthologs ( ferredoxin 2 and Oxidation Resistance 1 , OXR1 , respectively). We found that an allele in mtd consisting of a single-nucleotide polymorphism and an insertion of 101 base pairs associated with reduced lifespan under DR, but not AL, when compared to the wild-type allele (Fig. 1a , Supplementary Fig. 1a , Supplementary Data 2 ) [3] . In female flies, whole-body mtd RNAi driven by Act5c -GS- Gal4 (Fig. 1b ), but not Fdxh RNAi (Supplementary Fig. 1b ), resulted in DR-specific reduction in lifespan, suggesting the importance of mtd expression in DR-mediated longevity. In contrast, a strong null allele mtd-T2A-Gal4 strain ( mtd MI02920- T2A - Gal4 ) [5] caused lethality in development in approximately 99% of flies, and DR did not extend lifespan in the flies that survived to adulthood (Fig. 1c ). OXR1 loss in humans is associated with severe neurological defects and premature death [5] , whereas overexpression provides protection in a mouse model of amyotrophic lateral sclerosis [6] , but its cellular mechanism of action is unknown. OXR1 is often studied for its role in oxidative stress response [9] , [10] , but Wang et al. showed that its loss causes lysosomal dysfunction independent of oxidative stress [5] . Thus, identifying the mechanism of OXR1 will elucidate a valuable target for neurodegenerative diseases and aging. Fig. 1: mtd is upregulated allele-specifically by Traffic Jam (TJ) to extend lifespan under DR. a Alternate (Alt) mtd allele prevents lifespan extension by dietary restriction across DGRP strains. Dots represent median strain lifespan on AL (red) or DR (blue). Black bars represent mean across all strains. n = minimum 100 flies per strain. Data are presented as mean values across a single strain. Error bars represent mean value across all strains per condition +/- SD. b Conditional whole body mtd RNAi in adulthood reduces lifespan under DR conditions. Dashed lines = RNAi induced by RU486, solid lines = ethanol vehicle control. p value determined by log-rank test. c Homozygous mtd null allele dramatically reduces lifespan. Dashed lines = mtd MI02920 null allele strain, solid lines = w 1118 control. p value determined by log-rank test. d mtd mRNA in w 1118 fly head is upregulated by DR. Values normalized to AL. Samples taken after 7 days on AL or DR. n = 5 whole flies or abdomens, 50 heads, or 10 thoraces per biological replicate across minimum 3 independent experiments. Error bars represent mean value across replicates +/- SD. e Constitutively active pan-neuronal mtd RNAi in development and adulthood dramatically reduces lifespan compared to TRiP (empty vector) control. p value determined by log-rank test. f Conditional pan-neuronal mtd RNAi induced by RU486 in adulthood reduces lifespan only under DR conditions. p value determined by log-rank test. g Overexpression of human OXR1 , driven by mtd T2A -Gal4 rescues loss of mtd . Dashed lines = homozygous mtd MI02920 null allele flies, solid lines = heterozygous controls, and dashed with circles = homozygous mtd MI02920 null allele with mtd - Gal4 -driven hOXR1 OE . p value determined by log-rank test. h Conditional pan-neuronal overexpression of human OXR1 induced by RU486 in adulthood extends lifespan under DR conditions. p value determined by log-rank test. i Constitutively active overexpression of human OXR1 in development and adulthood extends lifespan. p value determined by log-rank test. j , DR increases mtd mRNA expression in heads of DGRP strains with the long-lived allele but not the short-lived allele. Samples taken after 7 days of AL or DR. n = 50 heads per replicate across 3 independent experiments. Error bars represent mean value across replicates +/- SD. k Schematic of LacZ reporter plasmid used for in vivo experiments in l – m . l LacZ staining is increased in whole brains from flies raised under DR transfected with cloned variant alleles from long-lived DGRP strains. Brains dissected after 7 days of AL or DR. n = 20 brains across 5 independent experiments. Error bars represent mean value across replicates +/- SD. m LacZ protein levels are increased in flies raised under DR transfected with long-lived variant allele reporter plasmid. Samples taken after 7 days of AL or DR. n = 20 heads per replicate across 5 independent experiments. Error bars represent mean value across replicates +/- SD. n Constitutively active pan-neuronal tj RNAi reduces mtd expression in fly heads. Values normalized to AL. n = 20 heads per replicate across 3 independent experiments. Error bars represent mean value across replicates +/- SD. o Conditional pan-neuronal tj RNAi induced in adulthood by RU486 reduces lifespan under DR. p value determined by log-rank test. For all figures, * p < 0.05, ** p < 0.005, *** p < 0.0005. Except where noted, all p values were calculated by two-sided t-test. 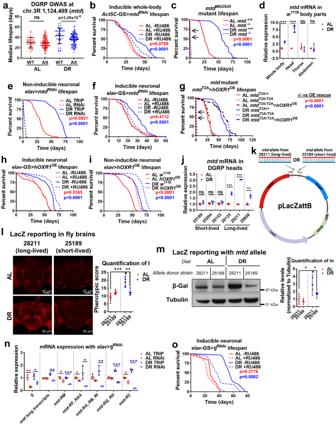Fig. 1:mtdis upregulated allele-specifically by Traffic Jam (TJ) to extend lifespan under DR. aAlternate (Alt)mtdallele prevents lifespan extension by dietary restriction across DGRP strains. Dots represent median strain lifespan on AL (red) or DR (blue). Black bars represent mean across all strains.n= minimum 100 flies per strain. Data are presented as mean values across a single strain. Error bars represent mean value across all strains per condition +/- SD.bConditional whole bodymtdRNAiin adulthood reduces lifespan under DR conditions. Dashed lines = RNAi induced by RU486, solid lines = ethanol vehicle control.pvalue determined by log-rank test.cHomozygousmtdnull allele dramatically reduces lifespan. Dashed lines =mtdMI02920null allele strain, solid lines =w1118control. p value determined by log-rank test.dmtdmRNA inw1118fly head is upregulated by DR. Values normalized to AL. Samples taken after 7 days on AL or DR.n= 5 whole flies or abdomens, 50 heads, or 10 thoraces per biological replicate across minimum 3 independent experiments. Error bars represent mean value across replicates +/- SD.eConstitutively active pan-neuronalmtdRNAiin development and adulthood dramatically reduces lifespan compared to TRiP (empty vector) control.pvalue determined by log-rank test.fConditional pan-neuronalmtdRNAiinduced by RU486 in adulthood reduces lifespan only under DR conditions.pvalue determined by log-rank test.gOverexpression of humanOXR1, driven bymtdT2A-Gal4 rescues loss ofmtd. Dashed lines = homozygousmtdMI02920null allele flies, solid lines = heterozygous controls, and dashed with circles = homozygousmtdMI02920null allele withmtd-Gal4-drivenhOXR1OE.pvalue determined by log-rank test.hConditional pan-neuronal overexpression of humanOXR1induced by RU486 in adulthood extends lifespan under DR conditions.pvalue determined by log-rank test.iConstitutively active overexpression of humanOXR1in development and adulthood extends lifespan.pvalue determined by log-rank test.j, DR increasesmtdmRNA expression in heads of DGRP strains with the long-lived allele but not the short-lived allele. Samples taken after 7 days of AL or DR.n= 50 heads per replicate across 3 independent experiments. Error bars represent mean value across replicates +/- SD.kSchematic of LacZ reporter plasmid used for in vivo experiments inl–m.lLacZ staining is increased in whole brains from flies raised under DR transfected with cloned variant alleles from long-lived DGRP strains. Brains dissected after 7 days of AL or DR.n= 20 brains across 5 independent experiments. Error bars represent mean value across replicates +/- SD.mLacZ protein levels are increased in flies raised under DR transfected with long-lived variant allele reporter plasmid. Samples taken after 7 days of AL or DR.n= 20 heads per replicate across 5 independent experiments. Error bars represent mean value across replicates +/- SD.nConstitutively active pan-neuronaltjRNAireducesmtdexpression in fly heads. Values normalized to AL.n= 20 heads per replicate across 3 independent experiments. Error bars represent mean value across replicates +/- SD.oConditional pan-neuronaltjRNAiinduced in adulthood by RU486 reduces lifespan under DR.pvalue determined by log-rank test. For all figures, *p< 0.05, **p< 0.005, ***p< 0.0005. Except where noted, allpvalues were calculated by two-sided t-test. Figure1kwas generated using BioRender (publishing license: KW266MCH0G). Figure 1k was generated using BioRender (publishing license: KW266MCH0G). Full size image DR induced a sevenfold increase in mtd mRNA expression in the head (Fig. 1d ). Neuronal mtd RNAi driven by the constitutively active elav - Gal4 induced developmental defects and severe lifespan reduction under both diets compared to TRiP (empty vector) control (Fig. 1e ), similar to whole-body loss of mtd . These phenotypes were not observed with intestine- or glia-specific mtd RNAi (Supplementary Fig. 1c, d ). To evaluate the impact of neuronal mtd RNAi with age, we used the conditional RU486-inducible elav -GS- Gal4 driver to induce a milder knockdown only in adulthood. This eliminated DR-mediated lifespan extension but did not alter lifespan on AL in females, whereas lifespan was reduced under both diets in males (Fig. 1f and Supplementary Fig. 1e, f ). There was no change in fecundity between RNAi and control flies (Supplementary Fig. 1g ). The TLDc domain in Mtd/OXR1 is responsible for neuroprotection [5] , [11] , so we overexpressed truncated human OXR1 containing this domain ( hOXR1 OE ) in neurons of flies that harbored the mtd null allele and observed a complete rescue of lifespan and DR response (Fig. 1g ). Neuronal hOXR1 OE in a wild-type background extended lifespan only under DR (Fig. 1h ), but also extended lifespan under AL conditions with stronger, constitutively active expression throughout life (Fig. 1i ). mtd expression was significantly increased across life in wild-type flies under DR, but this expression declined from day 7 to day 21 on both diets (Supplementary Fig. 1h ). Overall, these results demonstrate that neuronal mtd expression is elevated by DR, declines with age, and is necessary for DR-mediated lifespan extension and sufficient to extend lifespan regardless of diet. Traffic jam promotes mtd expression diet- and allele-specifically In the DGRP, strains with the long-lived allele had elevated mtd expression in the head under DR, unlike strains that harbor the short-lived allele (Fig. 1j ). Strains with the long-lived allele showed elevated expression of mtd transcripts that include exons 3′ of the variant only (Supplementary Fig. 1i ). However, transcripts with exons from both sides of the variant (“long transcripts”) showed elevated expression on DR regardless of allele (Supplementary Fig. 1j ). To validate the effects of these alleles, we cloned the allelic variant region into a LacZ reporter plasmid and transfected w 1118 wild-type flies (Fig. 1k ). Upon rearing under DR, flies with the long-lived allele showed elevated LacZ expression versus flies reared under AL and versus flies transfected with the short-lived allele (Fig. 1l, m ), suggesting that this genetic sequence influences nutrient-dependent changes in mtd expression. Using publicly available fly ChIP-seq data [12] , [13] , we found a significant binding signal at this locus for CCCTC-binding factor (CTCF) and Traffic jam (TJ) (Supplementary Fig. 1k ). Inducible neuronal ctcf RNAi increased mtd expression (Supplementary Fig. 1l ), whereas tj RNAi reduced expression of all mtd transcripts under DR (Fig. 1n ) and shortened lifespan specifically under DR (Fig. 1o ). We validated that TJ, the fly homolog of MAF, binds this locus via ChIP-PCR (Supplementary Fig. 1m ). In summary, we found that natural variants in mtd that show increased expression upon DR are regulated by TJ and are associated with lifespan extension upon DR, whereas CTCF represses mtd expression specifically under AL conditions, but that these effects only impact the shorter transcripts that are downstream of the variant site and TJ/CTCF binding site. mtd regulates the retromer complex To define the pathway affected by loss and gain of Mtd/OXR1, we analyzed gene ontology (GO) terms for the top 50 genes that show co-expression patterns similar to human OXR1 (Supplementary Data 4 ) [14] . These showed significant enrichment for protein trafficking from the endosome to the lysosome or recycling endosomes (Fig. 2a and Supplementary Data 5 ). Neuronal mtd RNAi increased levels of Atg8a-II (fly ortholog of LC3), a marker for autophagosome formation (Supplementary Fig. 2a ), consistent with the lysosomal accumulation phenotype observed in human fibroblasts and flies with OXR1 deficiency [5] . We co-stained human fibroblasts [5] for OXR1 and markers for vesicular transport organelles (lysosome, endosome, Golgi, endoplasmic reticulum, and mitochondria). OXR1 staining overlapped most with the endosomal marker RAB7 (Supplementary Fig. 2b ). As retromer dysfunction at the endosome causes lysosome dysfunction [15] as well as increased autophagosome formation [16] due to improper trafficking of endocytosed proteins and lipids, we hypothesized that OXR1 maintains retromer function. Neuronal mtd RNAi and tj RNAi significantly reduced the levels of retromer proteins (Fig. 2b and Supplementary Fig. 2c ). This was not due to reduced retromer gene transcription under mtd RNAi (Supplementary Fig. 2d ). Co-staining fly brains with antibodies against Mtd and retromer protein Vps35 with neuronal mtd RNAi also showed that Vps35 was reduced with mtd RNAi (Fig. 2c ). We also observed co-localization of Vps35 and Mtd in the brains of w 1118 control flies (Fig. 2d ), particularly in the optic lobes where OXR1 and the retromer have previously been shown to be relevant in flies [5] , [17] . We further determined that OXR1 interacts with VPS26A, VPS26B and VPS35 via co-immunoprecipitation in human fibroblasts (Fig. 2e ). Retromer maintenance is necessary for neuronal health [18] , [19] , and the loss of retromer proteins induces neurodegenerative disease progression [17] , [20] . Our results indicate that Mtd is involved in the maintenance of retromer function. Fig. 2: mtd interacts with the retromer complex and is required for retromer maintenance. a GO terms for the top 50 genes co-expressed with OXR1 show enrichment for endolysosomal network. Arranged by organelle and function. b , Vps35 and Vps26 levels are reduced in in heads with constitutively active pan-neuronal mtd RNAi . Quantification below. n = 5 heads per replicate per condition across minimum 3 independent experiments. Error bars represent mean value across replicates +/- SD. c Immunohistochemistry of brains from flies under constitutively active pan-neuronal mtd RNAi (bottom) show reduced Vps35 signal. Blue = DAPI, red = Vps35, green = Mtd. d Immunohistochemistry of w 1118 fly brains show co-localization of Mtd and Vps35. Image below merge is magnified from boxed region in whole-brain images. e Co-immunoprecipitation in lysates from human fibroblasts transduced with GFP alone or OXR1-GFP show interaction between OXR1 and retromer proteins VPS35, VPS26A, and VPS26B. IP immunoprecipitated sample, FT sample flow-through. For all figures, * p < 0.05, ** p < 0.005, *** p < 0.0005. All p values were calculated by two-sided t-test. 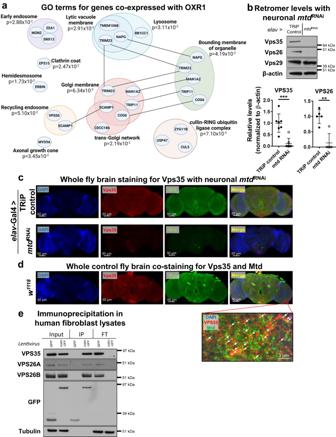Fig. 2:mtdinteracts with the retromer complex and is required for retromer maintenance. aGO terms for the top 50 genes co-expressed with OXR1 show enrichment for endolysosomal network. Arranged by organelle and function.b, Vps35 and Vps26 levels are reduced in in heads with constitutively active pan-neuronalmtdRNAi. Quantification below.n= 5 heads per replicate per condition across minimum 3 independent experiments. Error bars represent mean value across replicates +/- SD.cImmunohistochemistry of brains from flies under constitutively active pan-neuronalmtdRNAi(bottom) show reduced Vps35 signal. Blue = DAPI, red = Vps35, green = Mtd.dImmunohistochemistry ofw1118fly brains show co-localization of Mtd and Vps35. Image below merge is magnified from boxed region in whole-brain images.eCo-immunoprecipitation in lysates from human fibroblasts transduced with GFP alone or OXR1-GFP show interaction between OXR1 and retromer proteins VPS35, VPS26A, and VPS26B. IP immunoprecipitated sample, FT sample flow-through. For all figures, *p< 0.05, **p< 0.005, ***p< 0.0005. All p values were calculated by two-sided t-test. Figure2awas generated using BioRender (publishing license: YW266MCNQ5). Figure 2a was generated using BioRender (publishing license: YW266MCNQ5). Full size image Retromer stabilization rescues Mtd/OXR1 deficiency Next, we tested if enhancing retromer function rescues mtd RNAi phenotypes. Neuronal overexpression (by elav - Gal4 driver) of vps26 or vps35 rescued fly larval lethality (Fig. 3a ) and lifespan (Fig. 3b, c , Supplementary Fig. 3a ). Overexpression of vps35 also recovered the loss of lifespan extension by DR in mtd RNAi (Fig. 3c ). Moreover, pharmacological retromer stabilization with the compound R55 [21] also rescued developmental deformities (Fig. 3d ) and the shortened lifespan of flies with mtd RNAi (Fig. 3e ). R55 further extended lifespan under DR beyond that of control strains on DR (Fig. 3e, f ). However, simultaneous mtd RNAi and overexpression of autophagy genes Atg8 , Atg6 , or LAMP1 did not rescue developmental defects (Supplementary Fig. 3b ), suggesting that defects due to OXR1 deficiency are not due to a reduction in autophagic function. Fig. 3: Retromer stabilization rescues neuronal mtd / OXR1 deficiency in flies and human fibroblasts. a Retromer overexpression rescues developmental lethality induced by constitutively active neuronal mtd RNAi . n = at least 6 independent breeding chambers with 15 females to 5 males per chamber. Error bars represent mean value across replicates +/- SD. b Overexpression of vps26 rescues lifespan defects in flies with constitutively active neuronal mtd RNAi to the levels of flies under AL conditions. p value determined by log-rank test. c , Overexpression of vps35 rescues lifespan defects in flies with constitutively active neuronal mtd RNAi and restores DR-mediated lifespan extension. p value determined by log-rank test. d , R55 supplementation rescues developmental lethality induced by constitutively active neuronal mtd RNAi . n = at least 5 independent breeding chambers with 15 females to 5 males per chamber. Error bars represent mean value across replicates +/- SD. e 6 μM R55 supplementation throughout development and adulthood rescues lifespan defects in flies with constitutively active neuronal mtd RNAi and restores DR-mediated lifespan extension. p value determined by log-rank test. 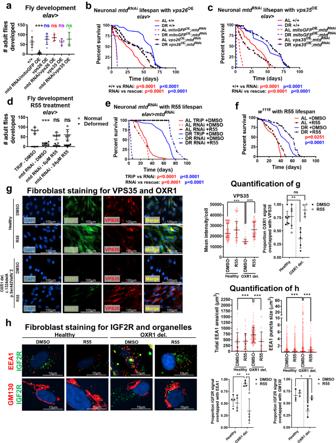Fig. 3: Retromer stabilization rescues neuronalmtd/OXR1deficiency in flies and human fibroblasts. aRetromer overexpression rescues developmental lethality induced by constitutively active neuronalmtdRNAi.n= at least 6 independent breeding chambers with 15 females to 5 males per chamber. Error bars represent mean value across replicates +/- SD.bOverexpression ofvps26rescues lifespan defects in flies with constitutively active neuronalmtdRNAito the levels of flies under AL conditions. p value determined by log-rank test.c, Overexpression ofvps35rescues lifespan defects in flies with constitutively active neuronalmtdRNAiand restores DR-mediated lifespan extension. p value determined by log-rank test.d, R55 supplementation rescues developmental lethality induced by constitutively active neuronalmtdRNAi.n= at least 5 independent breeding chambers with 15 females to 5 males per chamber. Error bars represent mean value across replicates +/- SD.e6 μM R55 supplementation throughout development and adulthood rescues lifespan defects in flies with constitutively active neuronalmtdRNAiand restores DR-mediated lifespan extension. p value determined by log-rank test.f6 μM R55 supplementation throughout adulthood only extends lifespan. p value determined by log-rank test.gHuman fibroblasts with a loss-of-function mutation inOXR1(c.132delA) have reduced VPS35 levels, which is rescued by 10 µM R55 supplementation. Blue = DAPI, green = OXR1, red = VPS35. Quantification on right.n= minimum 12 cells across minimum 4 independent experiments. Error bars represent mean value across replicates +/- SD.hImmunocytochemistry in human fibroblasts with loss-of-functionOXR1mutation show enlarged endosomes (EEA1, red in top row), increased number of endosomes, and inability to traffic IGF2R to Golgi (GM130, red in bottom row). Quantification on right.n= minimum 38 cells across minimum 3 independent experiments. Error bars represent mean value across replicates +/- SD. For all figures, *p< 0.05, **p< 0.005, ***p< 0.0005. Except where noted, all p values were calculated by two-sided t-test. 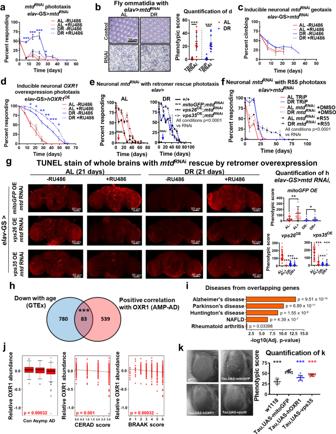Fig. 4: Retromer stabilization by R55 or OXR1 overexpression preserves vision and rescues tauopathy-related dysfunction. aFlies with RU486-induced neuronalmtdRNAiin adulthood show reduced responsiveness to light.n= minimum 50 flies per replicate across 4 independent experiments. Data represent mean value across replicates +/- SD.b, Flies with constitutively active pan-neuronalmtdRNAiin development have disordered eye ommatidia. Image quantification on right.n= eyes from minimum 11 fly heads per condition. Error bars represent mean value across replicates +/- SD.cNegative geotaxis is unaffected in flies with RU486-inducible neuronalmtdRNAi.n= at least 50 flies across 2 independent experiments. Data represent mean value across replicates +/- SD.dFlies with RU486-inducible pan-neuronal overexpression of humanOXR1in adulthood have improved phototaxis throughout the lifespan.n= at least 50 flies across 3 independent experiments. Data represent mean value across replicates +/- SD.eOverexpression ofvps26orvps35rescues loss of phototaxis in flies with constitutively active neuronalmtdRNAi. Dashed lines =mtdRNAi, dashed with solid circles =mtdRNAiwithvps26OE, dashed with open circles =mtdRNAiwithvps35OE. AL shown on left (red) and DR shown on right (blue).n= minimum 50 flies (except formtdRNAidue to larval lethality) per condition across 3 independent experiments. Data represent mean value across replicates +/- SD.fSupplementation with 6 μM R55 rescues loss of phototaxis in flies with constitutively active neuronalmtdRNAi.n= minimum 50 flies (except formtdRNAidue to larval lethality) per condition across 3 independent experiments. Data represent mean value across replicates +/- SD.gTUNEL stain for degeneration in aged fly brains is increased with RU486-inducible neuronalmtdRNAi(top row) but rescued by overexpression ofvps26(middle row) orvps35(bottom row). Flies were raised for 21 days under AL or DR with RU486 or vehicle control prior to sample collection. Quantification on right.n= minimum 17 fly brains per condition. Error bars represent mean value across replicates +/- SD.hVenn diagram demonstrating number of genes downregulated in GTEx dataset and proteins positively correlated with OXR1 from AMP-AD dataset. Overlap in the middle. Significance determined by Fisher Exact test.iAlzheimer’s disease, Parkinson’s disease, and Huntington’s disease are the most enriched diseases associated with the overlapping genes inh.pvalue adjusted for multiple testing.j, Correlation of OXR1 protein abundance with AD diagnosis (left), CERAD score (middle), and BRAAK score (right). Asymp = asymptomatic AD. n = 453 human brains. Box plots represent the median, 25th, and 75thpercentiles and whiskers represent the 5thand 95thpercentiles.k, Constitutively active neuronal overexpression of humanOXR1orvps35rescues degeneration induced by expression of mutantTaudriven in the fly eye with GMR promoter. Quantification of degenerative phenotype on right.n= eyes from minimum 11 fly heads per condition. Error bars represent mean value across replicates +/- SD. For all figures, *p< 0.05, **p< 0.005, ***p< 0.0005. Except where noted, allpvalues were calculated by two-sided t-test. f 6 μM R55 supplementation throughout adulthood only extends lifespan. p value determined by log-rank test. g Human fibroblasts with a loss-of-function mutation in OXR1 (c.132delA) have reduced VPS35 levels, which is rescued by 10 µM R55 supplementation. Blue = DAPI, green = OXR1, red = VPS35. Quantification on right. n = minimum 12 cells across minimum 4 independent experiments. Error bars represent mean value across replicates +/- SD. h Immunocytochemistry in human fibroblasts with loss-of-function OXR1 mutation show enlarged endosomes (EEA1, red in top row), increased number of endosomes, and inability to traffic IGF2R to Golgi (GM130, red in bottom row). Quantification on right. n = minimum 38 cells across minimum 3 independent experiments. Error bars represent mean value across replicates +/- SD. For all figures, * p < 0.05, ** p < 0.005, *** p < 0.0005. Except where noted, all p values were calculated by two-sided t-test. Full size image Retromer stabilization by R55 rescued VPS35 levels and VPS35 co-localization with OXR1 in human fibroblasts from patients with OXR1 mutations [5] (Fig. 3g ). The mutation in OXR1 also increased endosome size and number and impaired trafficking of mannose-6-phosphate receptor IGF2R from endosomes (EEA1 as marker) to the Golgi complex (GM130 as marker), all of which were rescued by treatment with 10 μM R55 (Fig. 3h ). R55 also significantly reduced the number of lysosomes in the OXR1 -deficient cells as well as localization of IGF2R with the lysosome (LAMP1 as marker) (Supplementary Fig. 3c, d ). Lysosomal protease Cathepsin B was significantly increased in OXR1 disease fibroblasts and further increased with R55 (Supplementary Fig. 3e ), despite the decreased lysosomal number in R55-treated cells. To further examine how lysosomal activity is impacted by OXR1-mediated retromer function, we compared LC3B-II levels in fibroblasts treated with the V-ATPase inhibitor bafilomycin, which blocks autophagy to demonstrate accumulated autophagosome pool size, to LC3B-II levels without bafilomycin, which represent steady-state pool size as LC3B-II is turned over during autolysosome formation [22] . OXR1 -deficient fibroblasts had significantly reduced basal LC3B-II compared to control cells, whereas blocking LC3B turnover with bafilomycin showed significantly greater LC3B-II levels than control cells, indicating increased LC3B turnover in the OXR1 -deficient cells. Treatment with 10 µM R55 increased the basal levels of LC3B-II in OXR1 -deficient fibroblasts, rescuing the LC3B-II levels compared to the deficient cells not treated with R55 (Supplementary Fig. 3f , additional statistics in Supplementary Data 1 ). Neuronal RNAi for vps26 and vps29 in adulthood reduced lifespan (Supplementary Fig. 3g ), with adulthood-specific vps26 RNAi reducing lifespan specifically under DR (Supplementary Fig. 3h ). Together, these results suggest that OXR1 is necessary for retromer function, and retromer stabilization rescues altered autophagic activity in human cells with OXR1 mutations and lifespan defects caused by mtd -deficiency in flies. Retromer stabilization rescues sensory decline and neurodegeneration induced by mtd RNAi To determine how mtd/OXR1 deficiency influences brain aging, we analyzed the transcriptomes of heads from younger (day 7) and older (day 21) flies with and without neuronal elav -GS- Gal4 -induced mtd RNAi through principal component analysis (PCA). Transcriptomes from older mtd RNAi DR flies grouped with older AL flies, suggesting that mtd RNAi accelerated transcriptional signatures towards older flies (Supplementary Fig. 4a and Supplementary Data 6 , 7 ). GO term analysis for mtd RNAi showed significant downregulation of genes associated with rhabdomere development and stimulus detection (Supplementary Fig. 4b and Supplementary Data 8 ), which have been implicated in retromer dysfunction in flies [17] , [23] . We observed delayed age-related visual decline upon DR, but this protective effect was abrogated by adulthood-specific neuronal mtd RNAi (Fig. 4a ). The ommatidia of the flies with constitutve RNAi were significantly more disordered than in TRiP empty vector controls (Fig. 4b ). We assessed negative geotaxis but observed no change in activity between flies with or without neuronal mtd RNAi , though activity was enhanced by DR (Fig. 4c ), suggesting an uncoupling of activity and eye degeneration as well as lifespan. To determine if accelerated sensory decline was restricted to the visual system, we tested chemotaxis throughout lifespan. Neuronal mtd RNAi under DR conditions induced more rapid decline in response to the attractant than DR controls, whereas flies under AL conditions were unaffected by RNAi (Supplementary Fig. 4c ), suggesting impaired neuronal signaling for two phenotypes commonly disrupted with age, vision and olfaction [24] , [25] . Pan-neuronal hOXR1 OE improved phototaxis throughout life under DR (Fig. 4d ). Retromer stabilization by vps26 OE or vps35 OE rescued phototaxis response in mtd RNAi flies (Fig. 4e ), as did treatment with 6 μM R55 (Fig. 4f ). We observed no significant changes in body mass, triglyceride levels, or starvation resistance upon inducible pan-neuronal induction of mtd RNAi (Supplementary Fig. 4d-f ). TUNEL staining in whole fly brains showed that flies reared on DR have reduced cellular apoptosis with age (21 days), but that inducible adult-specific mtd RNAi negates this benefit of DR. This elevated degeneration by mtd RNAi was rescued by overexpression of vps26 or vps35 in both diets (Fig. 4g , Supplementary Fig. 4g ). These results indicate that mtd and the retromer are necessary for delaying age-associated degeneration in the fly brain and sensory systems and attraction to stimuli, and that mtd does not affect triglyceride metabolism. Fig. 4: Retromer stabilization by R55 or OXR1 overexpression preserves vision and rescues tauopathy-related dysfunction. a Flies with RU486-induced neuronal mtd RNAi in adulthood show reduced responsiveness to light. n = minimum 50 flies per replicate across 4 independent experiments. Data represent mean value across replicates +/- SD. b , Flies with constitutively active pan-neuronal mtd RNAi in development have disordered eye ommatidia. Image quantification on right. n = eyes from minimum 11 fly heads per condition. Error bars represent mean value across replicates +/- SD. c Negative geotaxis is unaffected in flies with RU486-inducible neuronal mtd RNAi . n = at least 50 flies across 2 independent experiments. Data represent mean value across replicates +/- SD. d Flies with RU486-inducible pan-neuronal overexpression of human OXR1 in adulthood have improved phototaxis throughout the lifespan. n = at least 50 flies across 3 independent experiments. Data represent mean value across replicates +/- SD. e Overexpression of vps26 or vps35 rescues loss of phototaxis in flies with constitutively active neuronal mtd RNAi . Dashed lines = mtd RNAi , dashed with solid circles = mtd RNAi with vps26 OE , dashed with open circles = mtd RNAi with vps35 OE . AL shown on left (red) and DR shown on right (blue). n = minimum 50 flies (except for mtd RNAi due to larval lethality) per condition across 3 independent experiments. Data represent mean value across replicates +/- SD. f Supplementation with 6 μM R55 rescues loss of phototaxis in flies with constitutively active neuronal mtd RNAi . n = minimum 50 flies (except for mtd RNAi due to larval lethality) per condition across 3 independent experiments. Data represent mean value across replicates +/- SD. g TUNEL stain for degeneration in aged fly brains is increased with RU486-inducible neuronal mtd RNAi (top row) but rescued by overexpression of vps26 (middle row) or vps35 (bottom row). Flies were raised for 21 days under AL or DR with RU486 or vehicle control prior to sample collection. Quantification on right. n = minimum 17 fly brains per condition. Error bars represent mean value across replicates +/- SD. h Venn diagram demonstrating number of genes downregulated in GTEx dataset and proteins positively correlated with OXR1 from AMP-AD dataset. Overlap in the middle. Significance determined by Fisher Exact test. i Alzheimer’s disease, Parkinson’s disease, and Huntington’s disease are the most enriched diseases associated with the overlapping genes in h . p value adjusted for multiple testing. j , Correlation of OXR1 protein abundance with AD diagnosis (left), CERAD score (middle), and BRAAK score (right). Asymp = asymptomatic AD. n = 453 human brains. Box plots represent the median, 25 th , and 75 th percentiles and whiskers represent the 5 th and 95 th percentiles. k , Constitutively active neuronal overexpression of human OXR1 or vps35 rescues degeneration induced by expression of mutant Tau driven in the fly eye with GMR promoter. Quantification of degenerative phenotype on right. n = eyes from minimum 11 fly heads per condition. Error bars represent mean value across replicates +/- SD. For all figures, * p < 0.05, ** p < 0.005, *** p < 0.0005. Except where noted, all p values were calculated by two-sided t-test. Full size image mtd / OXR1 expression protects against neurodegenerative diseases and Alzheimer’s disease phenotypes To identify disorders associated with mtd / OXR1 , we determined proteins significantly downregulated in flies with neuronal mtd RNAi via data-independent acquisition mass spectrometry (q value < 0.05, Supplementary Data 9 , 10 ) [26] . This revealed significant enrichment for proteins involved in multiple human neurodegenerative diseases (Supplementary Data 11 ). We next analyzed -omics datasets from humans to learn more about the conserved nature of OXR1 in neurodegenerative diseases. We found an overlap of 83 genes between proteins with abundance levels that positively correlate with OXR1 (ρ > 0.30, Supplementary Data 12 ) from the Accelerating Medicines Partnership – Alzheimer’s Disease (AMP-AD) dataset [27] and genes affected by age from the Genotype-Tissue Expression (GTEx) project (Fig. 4h and Supplementary Data 13 ) [28] , [29] . KEGG pathway analysis for the genes, which overlapped between these datasets revealed significant enrichment for age-related neurodegenerative diseases, including Alzheimer’s, Huntington’s, and Parkinson’s diseases, (Fig. 4i and Supplementary Data 14 ) [30] . Retromer dysfunction has been associated with age-related neurodegenerative diseases that are protected by DR, including AD [31] , [32] , [33] , [34] , [35] , especially in trafficking cargo involved in disease progression [21] and maintaining synaptic function [36] . We therefore also analyzed human OXR1 and retromer-associated protein abundance using the AMP-AD dataset [37] . Lower levels of OXR1, VPS35, SNX5, and RAB7A were all significantly associated with AD diagnosis and poor memory and pathology scores (Fig. 4j and Supplementary Data 15 ). To determine if OXR1 or retromer overexpression could rescue phenotypes associated with AD and tau pathogenesis, we neuronally overexpressed hOXR1 or vps35 in flies with simultaneous GMR -driven pathogenic human Tau in the eyes. Flies with hTau OE alone showed rapid eye degeneration with no changes in overall tau levels, but neuronal hOXR1 OE or vps35 OE rescued this degeneration phenotype (Fig. 4k and Supplementary Fig. 4h–j ). These results demonstrate that the proteins in OXR1’s network play a critical and conserved role in humans and flies for brain aging and neurodegeneration. The widespread health and longevity benefits of DR are well-established, but the mechanisms by which DR mediates brain-specific functions are poorly understood. We previously showed in flies that DR elicits protective effects on lifespan and healthspan at least partially through distinct mechanisms [4] . While nutrient signaling pathways, such as TOR and ILS, are potential anti-aging pathways with roles in enhancing metabolism and burning fat [38] , the variability in response to DR across different individuals and in different tissues suggests there are still many molecular mechanisms that remain unelucidated [2] . While screening for DR-responsive mechanisms, we found a role for mtd / OXR1 in regulating neuronal health with age and in response to DR. Here, we showed that mtd / OXR1 is an essential gene for healthy brain aging. We found that alleles of mtd that are upregulated by DR are regulated by the transcription factor TJ, and that this expression is necessary for DR-mediated lifespan extension. Specifically, our form of DR primarily restricts overall protein intake. Under AL conditions, CTCF is upregulated, inhibiting the expression of mtd in flies. Thus, protein restriction allows for increased mtd expression. As elevated nutrient-related components have been linked to dysregulation of the retromer [39] , [40] , our work provides a genetic and molecular mechanism for this regulation. Mtd/OXR1 interacts with and maintains the retromer complex, and retromer stabilization rescues neurodegenerative and longevity defects induced by mtd / OXR1 deficiency. Our results show that OXR1 expression is necessary for DR-mediated lifespan extension, and that neuronal overexpression of OXR1 is sufficient for extending lifespan. While there is a large body of work demonstrating the benefits of DR, relatively few studies have detailed cellular mechanisms of DR on the brain. Our work presents a mechanism by which DR slows brain aging through the necessary action of OXR1 in maintaining the retromer. Retromer function is necessary for neuron survival [18] , [41] , [42] . Thus, elucidating novel retromer pathway components is valuable for promoting brain health, especially with aging. Retromer dysfunction has been associated with age-related neurodegenerative diseases that are protected by DR, specifically Alzheimer’s [31] , [43] , [44] and Parkinson’s diseases [17] , [45] , [46] , [47] , especially in trafficking cargo involved in disease progression, such as APP [21] and β-secretase [48] . Mtd/OXR1 provides a linchpin for this interactive relationship between retromer regulation and DR-mediated neuroprotection with age. Our findings with OXR1’s interaction with and regulation of retromer function resemble those of PLA2G6, which interacts directly with VPS26 and VPS35 [17] . PLA2G6 maintains the retromer to improve ceramide trafficking [17] . It remains to be explored by which mechanisms the components of the retromer are lost when OXR1 is absent. Our work also shows that the effects of OXR1 on the retromer complex influence the lysosomal phenotypes in cells from patients with OXR1 deficiencies, and this phenotype was rescued in patient cells supplemented with R55. These findings suggest that OXR1 is a necessary component to gain the benefits of autophagy, especially under DR conditions, and that these benefits are mediated by OXR1’s regulation of retromer function. An intriguing area of future research would be to determine if retromer proteins, such as VPS26 and VPS35, are degraded at an increased rate as a result of elevated autophagic function in instances of OXR1 loss. We further demonstrate that the OXR1 gene network, conserved in flies and humans, is an important target for brain aging and neurodegenerative diseases. Loss of mtd accelerated aging, neurodegeneration, and visual decline in flies, but this was rescued by retromer stabilization. Additionally, overexpression of OXR1 rescued age-related visual decline, neurodegeneration, and transgenically-induced tauopathy in a fly model. It remains to be observed which specific proteins or lipids are being mistrafficked, which result in neurodegeneration and reduction of lifespan with loss of OXR1 . It is also not yet known if variants in genes that regulate OXR1 might be associated with AD, as it seems that overall age-related decline in OXR1 is more likely the cause for its associations with neurodegeneration. Our proteomics data support this idea, as OXR1 declines significantly with age in AD patients. Our proteomics results in flies and humans also show enrichment for necessary components of synapses, and thus, future work could focus on understanding how changes in recycling influence neuronal function at the synapse. Additionally, OXR1 has been implicated through GWAS in regulating ceramide levels [49] . Ceramide buildup has previously been demonstrated as a cause of lifespan reduction under retromer dysfunction [17] , which could be an interesting area for future analysis. In all, our work implicates OXR1 and its network as a key regulators and potential therapeutic targets to slow aging and age-related neurodegenerative diseases across flies and humans. Genome-wide association analysis We used DGRP release 2 genotypes and FlyBase R5 coordinates for gene models. We used only homozygous positions and a minor allele frequency of ≥25% to ensure that the minor allele was represented by many observations at a given polymorphic locus [50] . We grouped the DGRP lines reared on a diet into a top 25 in-case group and a non-case group (>41 days median lifespan in DR conditions). The genotype distributions at each locus in these groups were compared via Fisher’s exact test using the SciPy.stats module in Python [51] . The genotypes were arranged in the contingency table configuration [[#CaseRefAllele/#CaseAltAllele], [#NonCaseRefAllele/#NonCaseAltAllele]]. Nominal p-values denoted as “ P value” in Supplementary Data 2 report the probability that the relative proportions of one variable are independent of the second variable. To avoid the potential for false positives at a given nominal cutoff owing to p-value inflation, we calculated false discovery rates via permutation as follows: for a given permutation i, we randomized phenotype values across DGRP lines, and assigned in- vs non-case designations on this permuted data set before we carried out Fisher’s exact tests for each marker in turn as above. We counted the number of markers n i that scored above a given p-value threshold t. We tabulated the false discovery rate at t as the ratio between the average n i across 10 permutations and the number of markers called at t in the real data. Gene expression analyses To determine gene expression in a normal system, we sampled 50 heads from mated females of w 1118 control strain after 1 week on an AL or DR diet. We isolated RNA using Zymo Quick RNA MiniPrepkit (R1054) (Zymo Research, Irvine, CA). For qRT-PCR, we used Superscript III Platinum SYBR Green One-Step qRT-PCR kit from Invitrogen, Carlsbad, CA (11736-051) and followed the manufacturer’s instructions with a Roche Lightcycler 480 II machine. Primers used are listed at the end of the Methods. To validate the effects of RNAi or mutation on gene expression, we collected 5 whole flies, 10 thoraces, 5 abdomens, or 50 heads after 1 week on AL or DR, depending on the body part being analyzed. We then isolated RNA from these samples and performed qRT-PCR on the perturbed genes as described above. RNA sequencing was performed by UC Berkeley QB3 Functional Genomics Laboratory, and reads were analyzed with the use of Bowtie2 read alignment package [52] , [53] . Two biological replicates per condition were used for RNA-seq analysis. Normalized reads counts are available in Supplementary Data Table S6 . Fly strains used in this study All flies were obtained from Bloomington Stock Center [54] , Vienna Drosophila Resource Center [55] , or FlyORF [56] and outcrossed six times to our lab control strains. Each line was mated and developed on a standard laboratory diet (1.5% yeast). At 2–3 days post-eclosion, unless otherwise noted, mated female progeny were transferred to AL (5.0% yeast extract) or DR (0.5% yeast extract) diet via CO 2 [57] . Living flies were transferred to fresh vials every other day, and dead flies were recorded until all flies were deceased. Flies were maintained in a 12-h light/dark cycle in a room maintained at 25 o C and 65% relative humidity [58] . A detailed list of fly strains used can be found at the end of the Methods section. Generation of LacZ transgenes The 0.41 kb mtd gene region fragment was generated by genomic PCR cloning of BglII-Xho I fragment into the BglII-XhoI site of pLacZattB. The genomic DNA was isolated from the short-lived strain BL25189, and PCR was performed with pLacZ primers (listed below). The 0.41 kb genomic PCR was generated using the same primers with genomic DNA isolated from the long-lived BL28211 strain as template. Transgenic insertion was performed by Rainbow Transgenic Flies (Camarillo, CA). The transgenes were verified by sequencing with pLacZ primers (listed below). The primers used for cloning and sequencing are listed below. Fly phenotyping We used the whole-body GeneSwitch driver Act5C -GS- Gal4 , neuron-specific inducible driver elav -GS- Gal4 , constitutively active elav - Gal4 driver, glia specific repo - Gal4 , or eye-specific rdgA - Gal4 for directed RNAi. 15 virgin driver females were mated with three transgene line males in four bottles containing a standard diet. At 2–3 days after progeny eclosion, mated females were sorted onto AL or DR media with 200 µM RU486 (final concentration) for inducible RNAi activation [58] , [59] or ethanol as vehicle control, and flies were maintained on these media for life. Body mass was measured in five replicates of three flies using a Radwag 82/220.X2 analytical balance. Flies were then frozen, and triglycerides were measured using Stanbio Triglycerides LiquiColor Test. Glucose was measured using Stanbio Liqui-UV Hexokinase kit. For both assays, absorbance was measured using SpectroMax M2 spectrophotometer. Starvation was performed by rearing adult flies for 10 days on an AL diet and then transferring to medium containing water and 1% agarose [58] . Flies were checked for deaths every 4 h until all flies were deceased. Pupariation rate was determined by mating flies and placing 60 resulting embryos on an AL diet. Number of pupae formed was recorded daily. For western blot analysis, fly heads were homogenized in TPER lysis buffer and protein concentrations were determined by BCA. Western blots were quantified using ImageQuant. List of antibodies is provided at the end of Methods section. Negative geotaxis was performed by placing flies in empty vial and counting proportion of flies that climbed 6 cm within 10 sec. Three replicates were performed per vial. Phototaxis was performed by placing flies in on end of a 30-cm horizontal tube and shining light at one end. The proportion of flies that had travelled to the last 10 cm at the other end was recorded [4] . Chemotaxis was performed by placing flies in a tube with one end containing a cotton plug saturated with 1 mL of 1-hexanol attractant, the other end with water. The proportion of flies in the segment with 1-hexanol after 30 sec was recorded [60] . Starvation, lifespan, phototaxis, chemotaxis, and geotaxis assays were performed with approximately 200 starting adult flies, except for constitutively active mtd RNAi and mtd mutant flies, since few flies reach development in these strains. Rough eye phenotype was analyzed using Flynotyper plug-in in Image J [61] . Images were taken with Olympus BX51 with 10X objective using fiber optics gooseneck microscope illuminator. 10-12 optical slices were taken and reconstitute using Zerenestacker (Zerene Systems, Richland, WA). Cell lines used in this study Patient cell lines were generated from skin biopsies and maintained in DMEM supplemented with 15% fetal bovine serum and 1% antibiotic cocktail [5] . Cells were maintained at 37 o C. Cells undergoing serum withdrawal were treated with medium without fetal bovine serum. The OXR1 deletion line is from a female patient. Cell lines and media are described at the end of the Methods. Fibroblast lysates Treatments with 10 μM R55 (Sigma-Aldrich #531084) were conducted for 48 h. Bafilomycin (100 nM, Cayman Chemical #11038) or DMSO control (Sigma Aldrich #276855) treatment was for 4 h prior to lysate collection. Lysates were collected with MPER lysis buffer and sonicated. Protein concentrations were determined by BCA. Western blots were quantified using ImageQuantTL. Co-immunoprecipitation Fibroblasts were transduced with lentivirus overexpressing OXR1-GFP (Origene RC231430L4) or GFP alone (Origene PS100093V) for 2 days at 2 MOI. Lysates were collected, homogenized, and sonicated in MPER lysis buffer with protease inhibitors. Protein G beads (GE Healthcare/Sigma 17061801) were washed in lysis buffer and samples were pre-cleared with beads for 4 h at 4 o C to remove non-specific interactions. Sample-bead slurry was spun down, sample was added to fresh tubes, and 5 μL anti-GFP primary antibody (sc-9996) was added to sample to incubate on inverting rocker overnight at 4 o C. Pre-washed beads were added to the sample-antibody solution and incubated for 4 h at 4 o C on inverting rocker. The sample was spun down, and unbound protein was collected as flowthrough sample (FT). Beads were washed 3 times with lysis buffer to ensure removal of unbound protein. The remaining sample and beads were incubated for 10 min at 95 o C with Invitrogen sample buffer and 1 M DTT for western blotting. LysoTracker Fibroblasts were plated in 8-well chamber slides and maintained for 48 h before supplementation with R55 or DMSO control for another 48 h. LysoTracker Deep Red (Thermo Fisher Cat#L12492) was diluted 1:2000 in medium for lysosome staining and Hoechst 33342 solution (Thermo Fisher Cat#62249) was diluted 1:1000 in medium for nuclear staining. Cells were incubated with stains for 30 min at 37 o C and then washed with medium and immediate imaged and analyzed using BioTek Cytation 5 Imaging Reader. Mean intensity of red fluorescence per nucleus was quantified. Immunocytochemistry After the treatments described above, cells were fixed in 4% paraformaldehyde in PBS. After three washes with PBS, cells were permeabilized using 0.1% Triton X-100 solution and blocked for 1 at room temperature with 1% bovine serum albumin and 5% donkey serum in PBS. Primary antibodies were diluted in blocking buffer, and cells were incubated overnight at 4 o C. After three washes with PBS, secondary antibodies (1:1000) were added and incubated for 1.5 h at room temperature. Slides were mounted with ProLong Gold antifade reagent with DAPI (Invitrogen Cat#P36931). Cells were imaged and analyzed using BioTek Cytation 5 Imaging Reader. List of antibodies used is provided at the end of the Methods section. Immunohistochemistry Adult Drosophila brains were dissected in PBS and immediately fixed in 4% PFA for 30 min. Post-fixation washes were done in PBS, and permeabilization was done in PT (PBS with 0.3% Triton X-100), three times for 30 min each. Blocking of tissues was done in permeabilization solution with 0.5% BSA. The brains tissue was labeled with primary antibodies (1:100) overnight in 4 o C, followed by three washes with PT solution. Secondary antibody incubation was for 2 h at room temperature. Tissues were then washed three times with PT and mounted with Fluoromount G mounting medium. All incubation steps were done with continuous mild shaking. Images were taken in Zeiss LSM 780 confocal microscope. List of antibodies used is provided at the end of the Methods section. TUNEL staining Adult Drosophila brains were dissected in PBS and immediately fixed in 4% PFA for 30 min. TUNEL staining was performed as per the manufacturer’s instruction with few changes (Roche #11684795910). Post-fixation washes were performed in PBS and permeabilization was performed in 0.1 % sodium citrate with 0.3% Triton X-100. Brains were incubated overnight with TUNEL solution and washed three times for 30 min each. Images were taken with Zeiss LSM 780 confocal microscope. Quantification was performed by counting TUNEL-positive cells per area. Proteomic analysis Heads from adult flies with or without pan-neuronal mtd RNAi were collected and flash frozen in liquid nitrogen in 5 replicates of at least 20 heads on the day of eclosion per replicate pool. Frozen heads from each condition/replicate were immersed in 100 μL of lysis buffer containing 4% SDS, 8 M urea, 200 mM triethylammonium bicarbonate (TEAB) at pH 8, 75 mM sodium chloride, 1 μM trichostatin A, 3 mM nicotinamide, and 1x protease/phosphatase inhibitor cocktail (Thermo Fisher Scientific, Waltham, MA). Lysates were subsequently homogenized for 2 cycles with a Bead Beater TissueLyser II (Qiagen, Germantown, MD) at 24 Hz for 3 min each, and further sonicated. Lysates were clarified by spinning at 15,700 x g for 15 min at 4 °C, and the supernatants containing the soluble proteins were collected. Protein concentrations were determined using a Bicinchoninic Acid Protein (BCA) Assay (Thermo Fisher Scientific, Waltham, MA), and subsequently 100 μg of protein from each sample were aliquoted. Samples were then solubilized using 4% SDS, 50 mM TEAB at a pH 8. Proteins were reduced using 20 mM DTT in 50 mM TEAB for 10 min at 50 °C followed by 10 min at RT, and proteins were subsequently alkylated using 40 mM iodoacetamide in 50 mM TEAB for 30 min at room temperature in the dark. Samples were acidified with 12% phosphoric acid to obtain a final concentration of 1.2% phosphoric acid, and diluted with seven volumes of S-Trap buffer (90% methanol in 100 mM TEAB, pH ~7). Samples were then loaded onto the S-Trap mini spin columns (Protifi, Farmingdale, NY), and spun at 4000x g for 10 s. The S-Trap columns were washed with S-Trap buffer twice at 4000x g for 10 s each. A solution of sequencing grade trypsin (Promega, San Luis Obispo, CA) in 50 mM TEAB at a 1:25 (w/w) enzyme:protein ratio was then added, and after a 1-hour incubation at 47 °C, trypsin solution was added again at the same ratio, and proteins were digested overnight at 37 °C. Peptides were sequentially eluted with 50 mM TEAB (spinning for 1 min at 1000x g ), 0.5% formic acid (FA) in water (spinning for 1 min at 1000x g ), and 50% acetonitrile (ACN) in 0.5% FA (spinning for 1 min at 4000x g ). After vacuum drying, samples were resuspended in 0.2% FA in water and desalted with Oasis 10-mg Sorbent Cartridges (Waters, Milford, MA). All samples were vacuum dried and resuspended in 0.2% FA in water at a final concentration of 1 μg/μL. Finally, indexed retention time standard peptides, iRT (Biognosys, Schlieren, Switzerland) [62] were spiked into the samples according to manufacturer’s instructions. The solvent system consisted of 2% ACN, 0.1% FA in water (solvent A) and 98% ACN, 0.1% FA in water (solvent B). Briefly, proteolytic peptides (2 μg) were loaded onto an Acclaim PepMap 100 C18 trap column with a size of 0.1 ×20 mm and 5 µm particle size (Thermo Fisher Scientific) for 5 min at 5 µL/min with 100% solvent A. Peptides were eluted on to an Acclaim PepMap 100 C18 analytical column sized as follows: 75 µm x 50 cm, 3 µm particle size (Thermo Fisher Scientific) at 0.3 µL/min using the following gradient of solvent B: 2% for 5 min, linear from 2% to 20% in 125 min, linear from 20% to 32% in 40 min, and up to 80% in 1 min, with a total gradient length of 210 min. Samples were analyzed by nanoLC-MS/MS in DIA mode [63] , [64] using a variable window isolation scheme [26] on the Orbitrap Eclipse Tribrid platform (Thermo Fisher Scientific, San Jose, CA). Samples were acquired in data-independent acquisition (DIA) mode. Full MS spectra were collected at 120,000 resolution (AGC target: 3e6 ions, maximum injection time: 60 ms, 350-1,650 m/z), and MS2 spectra at 30,000 resolution (AGC target: 3e6 ions, maximum injection time: Auto, NCE: 27, fixed first mass 200 m/z). The DIA precursor ion isolation scheme consisted of 26 variable windows covering the 350-1,650 m/z mass range with an overlap of 1 m/z [26] . DIA data were processed in Spectronaut v15 (version 15.1.210713.50606; Biognosys) using directDIA. Data were searched against the Drosophila melanogaster proteome with 42,789 protein entries (UniProtKB-TrEMBL), accessed on 12/07/2021. Trypsin/P was set as digestion enzyme and two missed cleavages were allowed. Cysteine carbamidomethylation was set as fixed modification, and methionine oxidation and protein N-terminus acetylation as variable modifications. Data extraction parameters were set as dynamic. Identification was performed using 1% precursor and protein q-value (experiment). Quantification was based on MS2 area, and local normalization was applied; iRT profiling was selected. Differential protein expression analysis was performed using a paired t-test, and p-values were corrected for multiple testing, specifically applying group wise testing corrections using the Storey method [65] . Protein groups with at least two unique peptides, q value < 0.05, and absolute Log2(fold-change) > 0.58 were considered to be significantly changed comparing mtd RNAi to TRiP empty vector control strain, and are listed in Supplementary Data Table S10 . Gene ontology analyses GO term analysis of Drosophila genes was performed using the set of all genes downregulated on day 14 from our RNA sequencing dataset. Analysis was performed using Gene Ontology enRIchment anaLysis and visuaLizAtion tool (GOrilla) and Process, Function, and Component analyses were all represented. For genes co-expressed with human OXR1, the top 50 genes from ARCHS [4] tool [14] were analyzed using ENRICHR GO Cellular Component 2021 Ontology list [30] . Statistics and reproducibility Significance of differences between survival curves was assessed by log rank test. p < 0.05 was considered statistically significant. Error bars represent SD across at least three biological replicates. Significant differences between experimental groups and controls are indicated by *. * p < 0.05, ** p < 0.005, *** p < 0.0005, determined by unpaired t test. nc = no change, ns = not significant. Significance for the Venn Diagram in Fig. 4h was calculated by Fisher’s Exact Test. Statistical analyses were calculated with GraphPad Prism 4. Additional statistical details, including starting n for each experiment, can be found in Supplementary Data 1 . Quantification of cell images was performed using BioTek imaging software. Statistics for genome-wide analyses were performed as previously stated. For Fig. 2c, d , each condition was tested with 20 fly brains with similar results. For Fig. 2e , experiment was repeated 3 times with similar results. Drosophila melanogaster strains used Strain Source ID number Drosophila Genetic Reference Panel strains Bloomington Drosophila Stock Center All DGRP strains Act5C-GS-Gal4 Driver (inducible, whole body) P{w[+mC]=Act5C(FRT.y[+])GAL4.Switch.PR}X, y[1] w[*] Bloomington Drosophila Stock Center #9431 Elav-GS-Gal4 Driver (inducible, neuronal) w1118; P{w[+mC]=elav-Switch.O}GSG301 Bloomington Drosophila Stock Center #43642 Elav-Gal4 Driver (non-inducible, neuronal) P{w[+mW.hs]=GawB}elav[C155] Bloomington Drosophila Stock Center #458 5966-GS-Gal4 (inducible, intestinal) +; 5966-GS Provided by lab of Dr. David Walker, University of California, Los Angeles N/A repo-Gal4 (non-inducible, glial) w[1118]; P{w[+m*]=GAL4}repo/TM3, Sb[1] Bloomington Drosophila Stock Center #7415 GMR-driven mutant Tau (non-inducible, eye), Elav-Gal4 (non-inducible, neuronal) P{w[+mW.hs]=GawB}elav[C155]; P{w[+mC]=GMR-htau/Ex}1.1 Bloomington Drosophila Stock Center #51360 w 1118 control strain Bloomington Drosophila Stock Center #5905 Transgenic RNAi Project (TRiP) empty vector control strain y[1] sc[*] v[1]; P{y[+t7.7] v[+t1.8] = VALIUM20-mCherry}attP2 Bloomington Drosophila Stock Center #35785 mtd RNAi y[1] sc[*] v[1]; P{TRiP.HMS01666}attP2/TM3, Sb[1] Bloomington Drosophila Stock Center #38519 mtd mutant y[1] w[*]; Mi{y[+mDint2]=MIC}mtd[MI02920]/TM3, Sb[1] Ser[1] Bloomington Drosophila Stock Center #76158 hOXR1 overexpression w1118; P{UAS-OXR1.HA}1 Bloomington Drosophila Stock Center #64104 hOXR1 overexpression w1118; P{UAS-OXR1.HA}4/TM3, Sb1 Bloomington Drosophila Stock Center #64105 Fdxh RNAi w1118; P{GD1274}v24497 Vienna Drosophila Resource Center #24497 CG15515 RNAi w1118; P{GD8577}v39872 Vienna Drosophila Resource Center #39872 tj RNAi y[1] sc[*] v[1]; P{TRiP.HMS01069}attP2 Bloomington Drosophila Stock Center #34595 TJ-GFP w[1118]; P33657Bac{y[+mDint2] w[+mC]=tj-GFP.FPTB}VK00033 Bloomington Drosophila Stock Center #66391 ctcf RNAi y[1] sc[*] v[1]; P{TRiP.GL00266}attP2 Bloomington Drosophila Stock Center #35354 ctcf RNAi y[1] v[1]; P{TRiP.HMS02017}attP40 Bloomington Drosophila Stock Center #40850 vps26 RNAi y[1] v[1]; P{TRiP.HMS01769}attP40 Bloomington Drosophila Stock Center #38937 vps29 RNAi y[1] v[1]; P{TRiP.HMJ21316}attP40 Bloomington Drosophila Stock Center #53951 vps35 RNAi y[1] sc[*] v[1] sev2[1]; P{TRiP.HMS01858}attP40 Bloomington Drosophila Stock Center #38944 Atg8 overexpression y[1] w[1118]; P{w[+mC]=UASp-GFP-mCherry-Atg8a}2 Bloomington Drosophila Stock Center #37749 hLAMP1 overexpression y[1] w[*]; PBac{y[+mDint2] w[+mC]=UAS-hLAMP1.HA}VK00033 Bloomington Drosophila Stock Center #86301 Atg1 overexpression y[1] w[*]; P{w[+mC]=UAS-Atg1.S}6 A Bloomington Drosophila Stock Center #51654 mitoGFP overexpression w[1118]; P{w[+mC]=UAS-mito-HA-GFP.AP}2/CyO Bloomington Drosophila Stock Center #8442 Cell lines and lentiviral vectors used Line Source ID F0062.1 Male human skin fibroblasts Healthy Provided by laboratory of Dr. Philippe Campeau, CHU Sainte Justine Research Center, Montreal, QC, Canada N/A F0342.1 Male human skin fibroblasts OXR1 mutation c.1324delA p.Ser44Valfs*2 Provided by laboratory of Dr. Philippe Campeau, CHU Sainte Justine Research Center, Montreal, QC, Canada N/A OXR1 (NM_001198533) Human Tagged ORF Clone pLenti-C-mGFP-P2A-Puro vector Origene RC231430L4 Lentiviral ORF control particles pLenti-C-mGFP-P2A-Puro Origene PS100093V Cell and fly media and additives used Dulbecco’s modification of Eagle’s medium, Corning VWR Cat#45000-304 Fetal bovine serum Life Technologies Cat#10082147 Penicillin-streptomycin Life Technologies Cat#15140122 Nutri-Fly Drosophila Agar, Gelidium Genesee Scientific Cat#66-104 Yellow Cornmeal Genesee Scientific Cat#62-100 Pure Cane Granulated Sugar C&H N/A Bacto yeast extract VWR Cat#90000-722 Saf instant yeast Rainy Day Foods Primers used mtd Forward Integrated DNA Technologies GAAGAAGACTCCAAGGAGCT mtd Reverse Integrated DNA Technologies CCCTATTTCTGCATCTAAGCG Bgl2 mtd promoter Fr Forward Integrated DNA Technologies GGAAGATCTGTGTACATATTGAATCAAATCAGC Xho1 mtd promoter Fr Reverse Integrated DNA Technologies TACGCTCGAGTTCTAGCCCTGTATCATACGG pLacZ attB Forward Integrated DNA Technologies GAAGTTATGCTAGCGGATCC pLacZ attB Reverse Integrated DNA Technologies GCGCCTCTATTTATACTCCGG tj Forward Integrated DNA Technologies GATTCTGGTGAACACATCTTCGG tj Reverse Integrated DNA Technologies TGGTGTGCGTAAGTCTGAGC ctcf Forward Integrated DNA Technologies GAGCGCCAACTCCAAGATCA ctcf Reverse Integrated DNA Technologies CCCATCGCCATACTCCTCAT mtd gene region Forward (for TJ ChIP) Integrated DNA Technologies GACCTCGAAAGAGTCGCCAT mtd gene region Forward (for TJ ChIP) Integrated DNA Technologies GATTCAGGGAATTGTGCGCC mtd-RM Forward Integrated DNA Technologies TGGAAGACCTCGAAAGAGT mtd-RM Reverse Integrated DNA Technologies CGAGTTCTCGGTTATCTACC mtd long transcripts Forward Integrated DNA Technologies TCGACTTGGACTCGCTCCG mtd long transcripts Reverse Integrated DNA Technologies TGGGTATGGTGGGCAATGAAG mtd-RF, RAA transcripts Forward Integrated DNA Technologies GAGAGCCGGATAATCCACGA mtd-RF, RAA transcripts Reverse Integrated DNA Technologies TCTCCATTGCGCCAGAAGAC mtd-RA, RB, RI transcripts Forward Integrated DNA Technologies AAAAACTTACGGCCACGCTG mtd-RA, RB, RI transcripts Reverse Integrated DNA Technologies TATTTCCCAGCGTCTCGTCG mtd-RQ, RH transcripts Forward Integrated DNA Technologies GCTGAATATGTTCGCCGCC mtd-RQ, RH transcripts Reverse Integrated DNA Technologies AAGCACTTGCAGAACATATAGAAAT mtd-RC transcript Forward Integrated DNA Technologies GAAGAGCGGAAGGCGTAGAG mtd-RC transcript Reverse Integrated DNA Technologies AAACGGCCAAGATGCCAAAC hOXR1 Forward Integrated DNA Technologies GGTTTGCTGTGCCACAAG hOXR1 Reverse Integrated DNA Technologies GGTTCTCTGGTATATTCGCCAG RpL32 Forward Integrated DNA Technologies TAAGCTGTCGCACAAATGG RpL32 Reverse Integrated DNA Technologies GGCATCAGATACTGTCCCT Act5C Forward Integrated DNA Technologies AAGTACCCCATTGAGCACGG Act5C Reverse Integrated DNA Technologies ACATACATGGCGGGTGTGTT vps26 Forward Integrated DNA Technologies GGTATCCGGCAAGGTGAACG vps26 Reverse Integrated DNA Technologies TTACCCCGGTCGTAGTACAGT vps29 Forward Integrated DNA Technologies CGAGAACCTGACGTATCCGG vps29 Reverse Integrated DNA Technologies AGGCCTCGAACTTGTACGTG vps35 Forward Integrated DNA Technologies GCCATTGGACTAGCGAGGAAG vps35 Reverse Integrated DNA Technologies AGCTCGTACAAATCCGTTTTCT tau Forward Integrated DNA Technologies CCATCATAAACCAGGAGGTGGCC tau Reverse Integrated DNA Technologies CTGTCTTGGCTTTGGCGTTCTC Antibodies and Stains Rabbit polyclonal anti-OXR1 Invitrogen Cat#PA5-72405 WB concentration: 1:500 Validated by RNAi Rabbit polyclonal anti-OXR1 abcam Cat#ab103042 ICC concentration: 1:100 Validated against human OXR1 mutation Goat polyclonal anti-VPS35 abcam Cat#ab10099 WB concentration: 1:500 ICC concentration: 1:100 Validated by KO (abcam) Rabbit polyclonal anti-VPS26A Proteintech Cat#12804-1-AP WB concentration: 1:500 Previously validated [66] Rabbit polyclonal anti-VPS26B Proteintech Cat#15915-1-AP WB concentration: 1:500 Validated by molecular weight Rabbit polyclonal anti-VPS29 Abcam Cat#ab236796 WB concentration: 1:500 Validated by KO (abcam) Mouse monoclonal anti-β-Galactosidase (LacZ) Promega Cat#Z3781 WB concentration: 1:500 IHC concentration: 1:100 Validated by molecular weight Rabbit polyclonal anti-LC3B Novus Biologicals Cat#NB100-2220 WB concentration: 1:150 Validated by KO (Novus Biologicals) Rabbit polyclonal anti-Atg8 Sigma-Aldrich Cat#ABC974 WB concentration: 1:500 Validated by molecular weight Mouse monoclonal anti-Cathepsin B [CA10] abcam Cat#ab58802 WB concentration: 1:500 Validated by molecular weight Rabbit polyclonal anti-GAPDH abcam Cat#ab9485 WB concentration: 1:500 Validated by molecular weight Rabbit polyclonal anti-β-actin Cell Signaling Cat#4967 WB concentration: 1:500 Validated by company (Cell Signaling) Mouse monocolonal anti-α-Tubulin [DM1A] Sigma-Aldrich Cat#T6199 WB concentration: 1:500 Validated by company (Sigma-Aldrich) Mouse monoclonal anti-Rab7 [EPR7589] abcam Cat#ab50533 WB concentration: 1:500 ICC concentration: 1:100 Validated by company (abcam) Mouse monoclonal anti-elav DSHB Cat#Elav-9F8A9 IHC concentration: 1:100 Validated by neuronal specificity Mouse monoclonal anti-EEA1 [G-4] Santa Cruz Biotechnology Cat#sc-137130 ICC concentration: 1:100 Validated by company (Santa Cruz Biotechnology) Mouse monoclonal anti-ATP5A [15H4C4] abcam Cat#ab14748 ICC concentration: 1:100 Validated by company (abcam) Mouse monoclonal anti-LAMP1 [H4A3] abcam Cat#ab25630 ICC concentration: 1:100 Validated by company (abcam) Mouse monoclonal anti-Calreticulin [FMC 75] abcam Cat#ab22683 ICC concentration: 1:100 Validated by company (abcam) Mouse polyclonal anti-GM130 abcam Cat#ab169276 ICC concentration: 1:100 Validated by company (abcam) Mouse monoclonal anti-GFP [B-2] Santa Cruz Biotech Cat#sc-9996 WB concentration: 1:500 Validated by molecular weight Mouse monoclonal anti-Tau [HT7] Invitrogen Cat#MN1000 WB concentration: 1:1000 Validated by molecular weight Sheep anti-Mouse IgG HRP-linked secondary Sigma Aldrich Cat#NXA931V WB concentration: 1:3000 Donkey anti-Rabbit IgG HRP-linked secondary Sigma Aldrich Cat#NA934V WB concentration: 1:3000 Mouse anti-Goat IgG HRP-conjugated secondary Santa Cruz Biotech Cat#sc-2354 WB concentration: 1:3000 Alexa Fluor 488 donkey anti-rabbit IgG (H + L) secondary Invitrogen Cat#A21206 ICC concentration: 1:500 Alexa Fluor 647 donkey anti-goat IgG (H + L) secondary Invitrogen Cat#A21447 ICC concentration: 1:500 Alexa Fluor 647 donkey anti-mouse IgG (H + L) secondary Invitrogen Cat#A21238 ICC concentration: 1:500 LysoTracker TM Deep Red Thermo Fisher Cat#L12492 Live cell imaging: 1:2000 Hoescht 33342 Solution Thermo Fisher Cat#62249 Live cell imaging: 1:1000 Reporting summary Further information on research design is available in the Nature Portfolio Reporting Summary linked to this article.